The prescience of paleoclimatology and the future of the Antarctic ice sheet 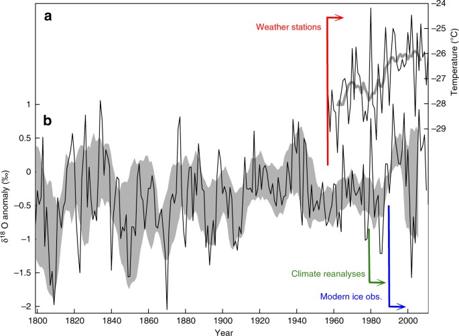Fig. 1 West Antarctic climate variability over the last 200 years.aMean-annual temperature data at the Byrd weather station.bOxygen isotope (δ18O) data from a collection of ice cores from the West Antarctic ice sheet. Gray shading shows decadal average with uncertainties. Vertical lines show the earliest year for which surface climate observations (red, 1957), climate reanalysis products (green, 1979) and spatially-complete geophysical ice-sheet observations (blue, ~1990) are available. Figure modified from Steig et al.18 The emerging view that the West Antarctic ice sheet is in the early stage of collapse owes as much to paleoclimatology as to contemporary observations.